Membrane deformation and scission by the HSV-1 nuclear egress complex The nuclear egress complex (NEC) of herpesviruses such as HSV-1 is essential for the exit of nascent capsids from the cell nucleus. The NEC drives nuclear envelope vesiculation in cells, but the precise budding mechanism and the potential involvement of cellular proteins are unclear. Here we report that HSV-1 NEC alone is sufficient for membrane budding in vitro and thus represents a complete membrane deformation and scission machinery. It forms ordered coats on the inner surface of the budded vesicles, suggesting that it mediates scission by scaffolding the membrane bud and constricting the neck to the point of scission. The inward topology of NEC-mediated budding in vitro resembles capsid budding into the inner nuclear membrane during HSV-1 infection and nuclear envelope vesiculation in NEC-transfected cells. We propose that the NEC functions as minimal virus-encoded membrane-budding machinery during nuclear egress and does not require additional cellular factors. Viruses are experts at remodelling cellular membranes—breaching them during cell entry or deforming them for budding. Viruses encode their own proteins and typically co-opt cellular machinery to achieve a specific task. Virus budding is a particularly complex process that involves membrane deformation around the viral capsid followed by the scission of the membrane at the neck of the viral bud. Many enveloped viruses use their own proteins for membrane deformation during bud formation and recruit components of the cellular endosomal sorting complex required for transport (ESCRT) machinery to achieve membrane scission during viral budding (reviewed in refs 1 , 2 , 3 ). Herpesviruses are a family of human pathogens that establish lifelong latent infections from which viruses periodically reactivate, causing a number of ailments. Reactivations are responsible not only for a significant disease burden but also for a high rate of new infections. During reactivation, progeny virions are assembled and released from the cell in a process called egress (reviewed in refs 4 , 5 ). As most other enveloped viruses, herpesviruses acquire their envelopes through budding. Uniquely, during egress, herpesvirus capsids bud twice. First, after being assembled in the nucleus, capsids bud into the inner nuclear membrane (INM) to form the perinuclear viral particles, which subsequently fuse with the outer nuclear membrane. The resulting cytosolic capsids then bud again into cytoplasmic membranes derived from Trans-Golgi Network [4] , [5] or the early endosomes [6] to be released from the cell by exocytosis. Cytoplasmic budding of herpesviruses is ESCRT-dependent [7] , [8] , similarly to cytoplasmic budding of most other enveloped viruses (reviewed in refs 1 , 2 , 3 ). By contrast, the nuclear budding is unique to herpesviruses [9] and is insensitive to the dominant-negative mutant of Vps4, suggesting that it is ESCRT-independent [8] . The nuclear egress complex (NEC) of herpesviruses, composed of conserved viral proteins UL31 and UL34, is essential for nuclear budding (reviewed in refs 4 , 9 ). Formation of the NEC is a prerequisite for proper localization of both UL31 and UL34 in the INM, as well as for recruitment of viral and cellular kinases for local dissolution of the nuclear lamina, for modification of host cell chromatin and for efficient nuclear egress of nucleocapsids (reviewed in refs 4 , 5 ). The NEC may reshape the INM around the capsid [10] , but the exact mechanism by which UL31 and UL34 accomplish this is unclear. The NEC is also sufficient to drive the vesiculation of the nuclear envelope in transfected cells [11] , [12] . But whether the NEC itself mediates membrane deformation and scission or recruits cellular proteins is unknown. Here, to determine the role of the NEC in nuclear membrane deformation and vesiculation, we use purified HSV-1 NEC lacking the TM helix of UL34, and characterize its interactions with model membranes. We show that the recombinant soluble HSV-1 NEC is a heterodimer that efficiently binds acidic liposomes and generates invaginations at the membrane-binding sites. Using fluorescent microscopy, we observe that the NEC drives membrane budding and scission of the intraluminal vesicles (ILVs) into giant unilamellar vesicles (GUVs) in vitro, in the absence of any other proteins. This result is recapitulated with NEC tethered to the membrane with an artificial anchor, confirming that the soluble NEC represents a useful model for studying the budding mechanism in vitro . Using cryoelectron microscopy, we find that the NEC assembles into ordered hexagonal coats on the inner surface of large unilamellar vesicles (LUVs). We propose that these NEC-coated LUVs represent the product of budding and scission, which the NEC accomplishes by a unique mechanism whereby a NEC coat scaffolds the membrane bud and constricts the neck to the point of scission. This scission mechanism differs from that of cellular ESCRT-III, which cleaves the neck from its exterior end [13] . Membrane deformation and scission induced by the soluble NEC in vitro are topologically equivalent to capsid budding during nuclear egress and to the INM vesiculation in cells transfected with the NEC. We propose that rapid assembly of an internal membrane-associated NEC coat is sufficient to drive membrane budding without the assistance of host factors. Our results suggest that the NEC can function as minimal virus-encoded membrane-budding machinery during nuclear egress and does not require additional cellular factors. HSV-1 NEC is a stable and properly folded heterodimer To determine if the NEC can drive membrane deformation in vitro in the absence of any other proteins, we expressed in Escherichia coli and purified several soluble versions of HSV-1 NEC composed of UL31 and UL34 proteins ( Fig. 1a,b , Supplementary Fig. 1a ). The following constructs were generated and expressed in E. coli : full-length HSV-1 UL31 (residues 1-306) and truncated UL31Δ50 (51-306), each bearing an amino-terminal tandem His6-SUMO tag, as well as HSV-1 UL34 constructs containing residues 1-246, 1-220 or 1-185 and an N-terminal GST tag ( Fig. 1a and Supplementary Fig. 1a ). To produce soluble NECs, all HSV-1 UL34 constructs used in this work lacked the entire transmembrane (TM) region and the 3-amino-acid tail facing the ER lumen. 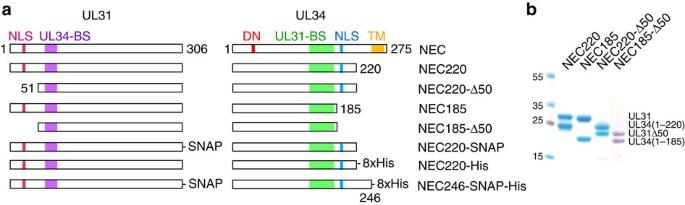Figure 1: Purification of soluble NECs. (a) Schematic view of HSV-1 UL31 and UL34 and constructs used here. NLS, nuclear localization sequence; BS, binding site; DN, dominant-negative mutation; TM, transmembrane region. (b) The purified NEC complexes are homogeneous as shown by 12% SDS–PAGE and Coomassie staining. Panels from two different gels are shown side by side (full gels are shown inSupplementary Fig. 7a). Figure 1: Purification of soluble NECs. ( a ) Schematic view of HSV-1 UL31 and UL34 and constructs used here. NLS, nuclear localization sequence; BS, binding site; DN, dominant-negative mutation; TM, transmembrane region. ( b ) The purified NEC complexes are homogeneous as shown by 12% SDS–PAGE and Coomassie staining. Panels from two different gels are shown side by side (full gels are shown in Supplementary Fig. 7a ). Full size image Initially, the full-length His6-SUMO-UL31 and three GST-UL34 constructs were expressed individually. Although GST-UL34 constructs could be purified, all three precipitated upon removal of the solubility tags, complicating biochemical and structural studies. His-SUMO-UL31 could not be purified to homogeneity and also precipitated upon removal of the solubility tag. This solubility problem was obviated when His6-SUMO-UL31 and GST-UL34 were coexpressed in E. coli or when the two proteins were expressed separately and the two lysates were mixed prior to purification. UL34(1-246) was prone to degradation and was not pursued further. Either UL34(1-220) or UL34(1-185) were coexpressed with UL31 or UL31Δ50, and the resulting NEC220, NEC185, NEC220-Δ50 and NEC185-Δ50 complexes were purified to homogeneity using a 4-step purification protocol that incorporated the removal of solubility tags ( Fig. 1b ). Although UL31 and UL34 need each other for solubility, they do not need to be coexpressed to form a complex; when the two proteins are expressed separately, a complex forms when the two lysates are mixed prior to purification. Thus, UL31 and UL34 probably do not need each other for folding. All four complexes, NEC220, NEC185, NEC220-Δ50 and NEC185-Δ50, are heterodimers judging by their elution volumes on size-exclusion chromatography ( Supplementary Fig. 1b ). For the NEC220, the stoichiometry was subsequently confirmed by multi-angle light scattering (MALS) ( Supplementary Fig. 1c ). The experimentally determined molecular weight of the NEC220, 58.92 kDa ( Supplementary Fig. 1c ), is consistent with a heterodimeric complex. Proper folding of NEC220 and NEC185 was further ascertained using circular dichroism (CD) spectroscopy ( Supplementary Fig. 1d,e ). Thus, the soluble NEC is a stably folded heterodimer. The NEC binds acidic lipids In both infected and transfected cells, the NEC localizes to the INM by means of the nuclear localization signal within UL31 and the carboxy-terminal TM anchor in UL34 (refs 14 , 15 , 16 ). We found that NEC220, lacking a TM anchor, bound model membranes as determined by coflotation and co-sedimentation ( Fig. 2 ). Membrane binding of NEC220 depended on lipid composition because nearly all NEC220 cofloated with LUVs containing 1-palmitoyl-2-oleoyl-sn-glycero-3-phosphocholine (PC), 1-palmitoyl-2-oleoyl-sn-glycero-3-phospho- L -serine (PS) and 1-palmitoyl-2-oleoyl-sn-glycero-3-phosphate (PA) in a 1:1:1 ratio but not with LUVs containing PC and cholesterol in a 1:1 ratio ( Fig. 2a ). Co-sedimentation assay with multilamellar vesicles (MLVs) was used to quantify binding [17] . The presence of at least 40% lipids containing anionic head groups (PS+PA) ( Fig. 2c ) was necessary for efficient binding, and liposomes with a PC:PS:PA=3:1:1 composition (40% acidic lipid) were used in subsequent experiments with the soluble NECs. The ~25% ‘background’ signal in the absence of liposomes is due to protein precipitation at the speed used in centrifugation; others have reported ‘background’ within that range in co-sedimentation assays [17] . 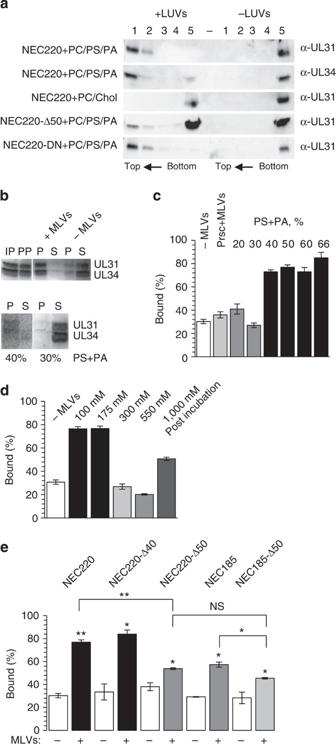Figure 2: The soluble NEC binds model membranes. (a) Membrane binding was determined using coflotation with 100 nm LUVs. Sucrose gradients, 5 ml in volume, were fractionated into five parts, from top (1) to bottom (5), and visualized by western blot using anti-UL31 or anti-UL34 antibodies (full western blots are shown inSupplementary Fig. 7b). (b) Membrane binding was quantified using co-sedimentation with MLVs and Coomassie staining (full gels are shown inSupplementary Fig. 7c). IP, input; PP, protein pellet; P, pellet; S, supernatant. (c) At least 40% of acidic lipid is required for NEC220 binding. As an additional negative control, liposomes were incubated with a PreScission protease (Prsc) that does not bind membranes. The ~30% ‘background’ signal in the absence of liposomes is due to protein precipitation at the speed used in centrifugation. (d) Interaction with MLVs depends on initial salt concentration. No binding was observed in the presence of NaCl concentrations higher than 175 mM. Addition of 1 M NaCl after complex formation did not abrogate the interaction. (e) Deletion of 50 but not 40 residues from the N terminus of UL31 reduces binding. The NEC185 binds worse than the NEC220 and combination of both truncations (NEC185-Δ50) lowers the binding affinity further. Experiments in c–e were done in triplicate, and the reported values represent averages of the results of three individual experiments. Error bars represent the s.e. of measurement. The statistical analysis used is the Student’st-test. One asterisk indicatesP-values smaller than 0.05 and two asterisks indicateP-values smaller than 0.005. The asterisks above each sample represent the significance compared with the background, whereas the asterisks above each line represent the significance between these two samples after subtracting the individual background levels. Figure 2: The soluble NEC binds model membranes. ( a ) Membrane binding was determined using coflotation with 100 nm LUVs. Sucrose gradients, 5 ml in volume, were fractionated into five parts, from top (1) to bottom (5), and visualized by western blot using anti-UL31 or anti-UL34 antibodies (full western blots are shown in Supplementary Fig. 7b ). ( b ) Membrane binding was quantified using co-sedimentation with MLVs and Coomassie staining (full gels are shown in Supplementary Fig. 7c ). IP, input; PP, protein pellet; P, pellet; S, supernatant. ( c ) At least 40% of acidic lipid is required for NEC220 binding. As an additional negative control, liposomes were incubated with a PreScission protease (Prsc) that does not bind membranes. The ~30% ‘background’ signal in the absence of liposomes is due to protein precipitation at the speed used in centrifugation. ( d ) Interaction with MLVs depends on initial salt concentration. No binding was observed in the presence of NaCl concentrations higher than 175 mM. Addition of 1 M NaCl after complex formation did not abrogate the interaction. ( e ) Deletion of 50 but not 40 residues from the N terminus of UL31 reduces binding. The NEC185 binds worse than the NEC220 and combination of both truncations (NEC185-Δ50) lowers the binding affinity further. Experiments in c–e were done in triplicate, and the reported values represent averages of the results of three individual experiments. Error bars represent the s.e. of measurement. The statistical analysis used is the Student’s t -test. One asterisk indicates P -values smaller than 0.05 and two asterisks indicate P -values smaller than 0.005. The asterisks above each sample represent the significance compared with the background, whereas the asterisks above each line represent the significance between these two samples after subtracting the individual background levels. Full size image Membrane binding of the NEC220 was sensitive to NaCl concentrations above 175 mM when NaCl was added along with liposomes ( Fig. 2d ). But, NEC220 binding to liposomes was less sensitive to the presence of high salt when the protein/liposome mix was incubated for 30 min prior to the addition of 1 M NaCl: nearly all of the NEC220 cofloated with liposomes ( Fig. 2a ) and most of NEC220 co-sedimented with liposomes ( Fig. 2d ). Salt sensitivity of the NEC220 binding suggests that the recruitment of NEC220 to liposomes is driven by electrostatic interactions. After the initial interaction, the dissociation was less sensitive to high salt, probably due to other types of interactions dominating the association with the membrane. Two regions within the NEC220 are necessary for membrane binding Membrane interactions of the NEC220 require residues 1-50 of UL31 and residues 186-220 of UL34 ( Fig 2a,e ). Removal of either region individually reduced membrane binding while the combined removal of both regions reduced binding even further ( Fig. 2e ). Residues 1-50 of UL31 are poorly conserved and are not predicted to adopt any regular secondary structure. While deletion of residues 1-50 reduced binding substantially ( Fig. 2e ), deletion of residues 1-40 did not affect binding, indicating that residues 41-50 in UL31 are necessary for membrane interaction. Binding of NEC to membrane relies on electrostatic interactions, and basic residues, lysines or arginines, are frequently found to interact with membranes electrostatically. Region 41-50 contains four basic residues that frame the hydrophobic LPP sequence ( Supplementary Fig. 2a ). To explore the relative contributions of these residues to membrane binding, we generated mutants R41S/K42S, R49S/K50S, R41S/K42S/R49S/K50S, L44S/P45T/P46T and L44S/A48S and tested them in a co-sedimentation assay ( Supplementary Fig. 2a ). None of the mutations impaired membrane binding, and we conclude that residues 41-50 probably do not interact with the membrane directly. The NEC causes membrane deformation and scission in vitro To investigate the membrane-deforming activity of the NEC220, we used an in vitro fluorescent assay with GUVs that has been previously used to image membrane deformation, budding and scission [13] , [17] , [18] , [19] . Red fluorescent GUVs were made by incorporating 2% POPE-Atto594. To visualize protein, we produced and purified the NEC220–SNAP complex, in which UL31 contained a C-terminal SNAP tag, and labelled it with green fluorescent dye SNAP Surface 488. In the absence of protein, the GUVs were mostly spherical with a diameter of ~3–15 μm ( Fig. 3a ). Immediately after being added to the GUVs, NEC220-SNAP bound to the vesicles, and we detected many deformed, rather than spherical, vesicles with flat sides or with invaginations at the sites of bound NEC220-SNAP ( Fig. 3b ). Thus, binding of soluble NEC220-SNAP to membranes induced negative, or inward, curvature. Moreover, after longer incubations, we frequently observed protein-covered membranes inside the GUVs, suggesting that the NEC220-SNAP can induce budding into the GUV lumen ( Fig. 3b ). 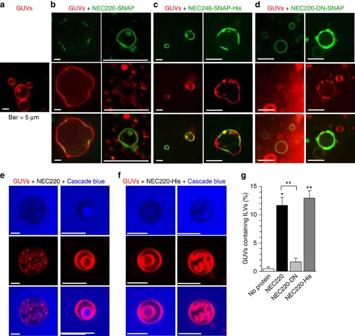Figure 3: NEC220 binding to GUVs drives membrane invagination and scission. GUVs containing 2% DOPE-ATTO594 (red) were visualized alone or in the presence of the NEC220-SNAP labelled with SNAP Surface 488 (green). (a) Free GUVs are spherical. (b) Upon addition of the NEC220, membrane invaginations and protein-bound ILVs inside intact GUVs were observed. Images show membrane invaginations wherever the NEC220 is bound. (c) GUVs containing a Nickel-chelated lipid were used with NEC246-His to mimic the membrane anchor. These GUVs were less acidic, but a similar scenario as with the soluble NEC220 could be observed. Wherever the protein is bound, the GUVs are flattened. (d) In the presence of NEC220-DN, GUVs are mostly spherical even after prolonged incubation. (e,f) When GUVs (red) were sequentially incubated with non-permeable fluorescent dye Cascade Blue and the unlabelled NEC220 or His-tagged NEC220, ILVs containing Cascade Blue were observed. (g) Quantification of these vesicles show that 12% of all GUVs contain ILVs when NEC220 was added, whereas there are no Cascade Blue-filled ILVs in the absence of any protein or in the presence of NEC220-DN. NEC220-His shows a similar behaviour with less acidic GUVs (13% ILVs) as the soluble NEC220. The reported values represent averages of the results of at least two individual experiments. Error bars represent the s.e. of measurement from at least two individual experiments, with a count of at least 67 GUVs per sample and experiment. The number of vesicles counted in total are as follows: no protein (104, 111), NEC220 (83, 75, 119), NEC220-DN (77, 136), NEC220-His (67, 86, 109). The statistical analysis used is the Student’st-test. One asterisk indicatesP-values smaller than 0.01. Two asterisks indicateP-values smaller than 0.005. Asterisks located above the black line indicate significance between these samples and asterisks above each data point indicate the significance compared with ‘no protein’ control. Figure 3: NEC220 binding to GUVs drives membrane invagination and scission. GUVs containing 2% DOPE-ATTO594 (red) were visualized alone or in the presence of the NEC220-SNAP labelled with SNAP Surface 488 (green). ( a ) Free GUVs are spherical. ( b ) Upon addition of the NEC220, membrane invaginations and protein-bound ILVs inside intact GUVs were observed. Images show membrane invaginations wherever the NEC220 is bound. ( c ) GUVs containing a Nickel-chelated lipid were used with NEC246-His to mimic the membrane anchor. These GUVs were less acidic, but a similar scenario as with the soluble NEC220 could be observed. Wherever the protein is bound, the GUVs are flattened. ( d ) In the presence of NEC220-DN, GUVs are mostly spherical even after prolonged incubation. ( e , f ) When GUVs (red) were sequentially incubated with non-permeable fluorescent dye Cascade Blue and the unlabelled NEC220 or His-tagged NEC220, ILVs containing Cascade Blue were observed. ( g ) Quantification of these vesicles show that 12% of all GUVs contain ILVs when NEC220 was added, whereas there are no Cascade Blue-filled ILVs in the absence of any protein or in the presence of NEC220-DN. NEC220-His shows a similar behaviour with less acidic GUVs (13% ILVs) as the soluble NEC220. The reported values represent averages of the results of at least two individual experiments. Error bars represent the s.e. of measurement from at least two individual experiments, with a count of at least 67 GUVs per sample and experiment. The number of vesicles counted in total are as follows: no protein (104, 111), NEC220 (83, 75, 119), NEC220-DN (77, 136), NEC220-His (67, 86, 109). The statistical analysis used is the Student’s t -test. One asterisk indicates P -values smaller than 0.01. Two asterisks indicate P -values smaller than 0.005. Asterisks located above the black line indicate significance between these samples and asterisks above each data point indicate the significance compared with ‘no protein’ control. Full size image To confirm that the NEC220 can mediate budding and, perhaps, even scission, non-permeable fluorescent dye Cascade Blue was added to the aqueous phase of the GUV sample. Shortly after addition of NEC220, we detected ILVs containing Cascade Blue inside the GUVs ( Fig. 3e ). Although ILVs were occasionally observed within the GUVs in the absence of NEC220 as a side effect of the GUV formation procedure ( Fig. 3a ), virtually no Cascade Blue-filled vesicles were observed in the absence of the NEC220 ( Fig. 3g ). Cascade Blue dye cannot penetrate the membrane; therefore, the presence of dye-filled ILVs inside the GUVs confirms that NEC220 mediates membrane budding. Moreover, ILVs were moving rapidly within the boundaries of the GUVs ( Supplementary Movie 1 ) indicating that scission had taken place [18] . These observations show that the NEC220 alone is sufficient for mediating not only budding but also scission of the model membranes. In the presence of the NEC220, ILVs formed rapidly, within 5–30 min, unlike in the presence of NEC220-SNAP, and we hypothesize that the SNAP tag in NEC220-SNAP impaired membrane budding. All subsequent budding experiments with Cascade Blue were carried out with NEC220 lacking SNAP tag. To determine whether membrane budding by the soluble NEC220 could model membrane budding mediated by the membrane-anchored NEC, we produced the soluble NEC complexes in which UL34 contained a C-terminal octa-histidine tag ( Fig. 1 ). Histidine tags mimic membrane anchors by anchoring proteins to liposomes containing Ni-chelating lipids [20] . NEC246-SNAP-His, in which UL31 contained a C-terminal SNAP tag while UL34 contained a C-terminal His tag, was used to monitor membrane binding and deformation. NEC220-His, in which UL34 contained a C-terminal His tag, was used to monitor ILV formation in the presence of Cascade Blue. Although the nuclear envelope is rich in PC and contains both PS and PA [21] , [22] , the liposomes used thus far had a relatively high acidic lipid content of 40%. We hypothesized that the requirement for such high acidic lipid content could be due to the lack of the TM anchor and that membrane-anchored NEC may be less reliant on acidic lipids for membrane interaction. In the experiments with the His-tagged NECs, we used GUVs containing 18% acidic lipid (57% PC, 13% PE, 9% PS, 9% PA, 5% cholesterol, 5% DGS-NTA, 2% PE-ATTO594), which mimicked the nuclear envelope composition more accurately. We found that like soluble NEC220-SNAP, membrane-anchored NEC246-SNAP-His generated negative curvature upon binding to the GUVs containing 18% acidic lipid ( Fig. 3c ). Moreover, NEC220-His also mediated ILV formation into these less acidic GUVs ( Fig. 3f ). To compare the budding efficiency of the NEC220 and NEC220-His, we quantified the number of GUVs containing Cascade Blue-filled ILVs ( Fig. 3g ). No Cascade Blue-filled ILVs were observed in the absence of protein, even after prolonged incubation ( Fig. 3g ). Both soluble and membrane-anchored NECs mediated budding with similar efficiency, ~12–13%. Increasing the protein concentration fourfold resulted in clusters or aggregates of small vesicles ( Supplementary Fig. 3 ), which were also observed after long incubations at lower NEC concentrations. These aggregates probably represent budding carried to completion when no ‘mother’ vesicles remain. Our results show that the budding of the less acidic GUVs by the membrane-tethered NEC220-His is comparable with the budding of the acidic GUVs by soluble NEC220. This result establishes that the soluble NEC220 in combination with acidic liposomes recapitulates membrane budding by membrane-anchored NEC and can be used as a model for studying the budding mechanism in vitro . The NEC forms coats on the inside of budded LUVs To visualize NEC bound to model membranes, LUVs, we used cryoelectron microscopy and tomography. Without the NEC, LUVs, which ranged in diameter between 300–800 nm appeared as smooth, spherical and mostly unilamellar liposomes, although some multilamellar liposomes were also present ( Fig. 4a and Supplementary Fig. 4a ). In the presence of the NEC220, the LUVs appeared to be smaller, with diameters of 100–300 nm, and the majority of the LUVs (over 50%) were coated with ordered protein arrays on the inside ( Figs 4a,b , 5a and Supplementary Figs 4,5 ). The NEC220 is unlikely to cross membranes, and we infer that the LUVs containing the inner NEC220 coats ( Figs 4b , 5e ) are the result of membrane budding and scission ( Fig. 4d ). This inference is supported by the observation that none of the LUVs in the presence of protein were as large as the LUVs alone ( Fig. 4a and Supplementary Fig. 4 ). 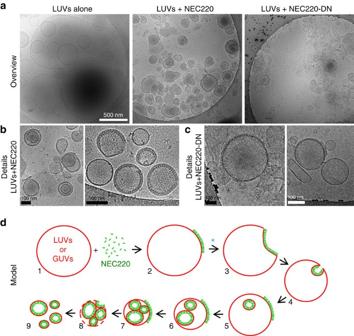Figure 4: The NEC220 but not the NEC220-DN mutant forms ordered arrays on the inner surface of the LUVs. (a) Representative cryoelectron micrographs of LUVs (400 and 800 nm) alone, in the presence of NEC220 or in the presence of NEC220-DN. (b) The NEC220 forms ordered arrays on the inner surface of the LUVs. (c) The NEC220-DN mutant forms clusters of spikes mainly on the outer surface of the LUVs. (d) A model of how membrane binding and oligomerization of the NEC leads to membrane invagination and scission, based on fluorescence and cryoelectron microscopy. Presumed steps are numbered. The ‘mother’ vesicle eventually breaks down, releasing intact vesicles coated with the NEC on the inside. The NEC220-DN mutant does not proceed beyond step 2 (blue asterisk). Figure 4: The NEC220 but not the NEC220-DN mutant forms ordered arrays on the inner surface of the LUVs. ( a ) Representative cryoelectron micrographs of LUVs (400 and 800 nm) alone, in the presence of NEC220 or in the presence of NEC220-DN. ( b ) The NEC220 forms ordered arrays on the inner surface of the LUVs. ( c ) The NEC220-DN mutant forms clusters of spikes mainly on the outer surface of the LUVs. ( d ) A model of how membrane binding and oligomerization of the NEC leads to membrane invagination and scission, based on fluorescence and cryoelectron microscopy. Presumed steps are numbered. The ‘mother’ vesicle eventually breaks down, releasing intact vesicles coated with the NEC on the inside. The NEC220-DN mutant does not proceed beyond step 2 (blue asterisk). 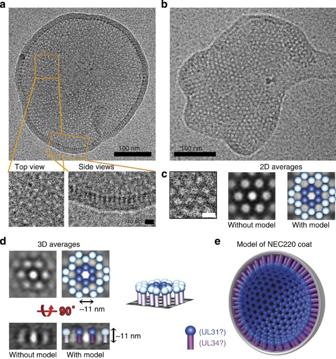Figure 5: NEC220 forms hexagonal honeycomb arrays on LUVs. (a) Cryo-EM image of a representative vesicle with close-up views of two types of observed arrays, rings arranged in a honeycomb pattern and ‘fences’. (b) A membrane patch from a broken LUV shows a single-layer NEC220 array. (c) A close-up view of the hexagonal array. Two-dimensional averaging enhances the sixfold symmetry. A model of NEC220 has been placed over the electron densities to highlight the protein densities. NEC220 spike is depicted as a magenta cylindrical stem topped with a blue sphere. (d) Three-dimensional-averaged cryo-EM images in top and side views are shown side by side with models of NEC220 placed over the electron densities to highlight the protein densities. A model of a section of the NEC220 hexagonal array in a slanted view is also shown. (e) The model of the membrane-bound inner NEC220 coat. UL31 has been tentatively assigned to the blue ‘sphere’ part of the spike on the basis of the cross-linking data. UL34 has been tentatively assigned to the ‘stem’ part because in the full-length NEC, UL34 anchors the complex to the membrane. These assignments are approximate and are not based on any direct structural data. The precise arrangement of UL31 and UL34 within the membrane-bound NEC spike is as yet unknown. Full size image Figure 5: NEC220 forms hexagonal honeycomb arrays on LUVs. ( a ) Cryo-EM image of a representative vesicle with close-up views of two types of observed arrays, rings arranged in a honeycomb pattern and ‘fences’. ( b ) A membrane patch from a broken LUV shows a single-layer NEC220 array. ( c ) A close-up view of the hexagonal array. Two-dimensional averaging enhances the sixfold symmetry. A model of NEC220 has been placed over the electron densities to highlight the protein densities. NEC220 spike is depicted as a magenta cylindrical stem topped with a blue sphere. ( d ) Three-dimensional-averaged cryo-EM images in top and side views are shown side by side with models of NEC220 placed over the electron densities to highlight the protein densities. A model of a section of the NEC220 hexagonal array in a slanted view is also shown. ( e ) The model of the membrane-bound inner NEC220 coat. UL31 has been tentatively assigned to the blue ‘sphere’ part of the spike on the basis of the cross-linking data. UL34 has been tentatively assigned to the ‘stem’ part because in the full-length NEC, UL34 anchors the complex to the membrane. These assignments are approximate and are not based on any direct structural data. The precise arrangement of UL31 and UL34 within the membrane-bound NEC spike is as yet unknown. Full size image We have not detected individual stages in membrane budding in the cryo-EM experiment instead observing only the coated LUVs that are likely the result of budding and scission ( Fig. 4d ). We conclude that budding into the LUVs occurs rapidly, which is consistent with the rapid formation of the ILVs in the Cascade Blue experiment ( Fig. 3e ). We also observed that the protein-coated LUVs were frequently found on their own instead of within the lumen of large LUVs. We propose that the excess of protein results in multiple budding events such that the ‘mother’ LUV eventually breaks down, releasing intact vesicles coated with the NEC on the inside ( Fig. 4d ). The NEC forms hexagonal honeycomb coats NEC220 formed ‘fences’ of spikes emanating from the membrane towards the vesicle interior in side views of the membrane and arrays of rings arranged in a hexagonal ‘honeycomb’ pattern in top (or planar) views of the membrane ( Fig. 5a , Supplementary Fig. 5 and Supplementary Movies 2,3 ). Occasionally, we also observed patches of a flattened membrane containing a single layer of NEC220 molecules arranged in a highly regular hexagonal honeycomb array in the top views ( Fig. 5b ). These patches could originate from either NEC220 interacting with flat membrane fragments or from NEC220-coated LUVs damaged during freezing of cryo samples. Measurements of 2D cryo-EM images ( Fig. 5a ) suggested and 3D tomographic reconstructions ( Fig. 5d , Supplementary Fig. 5 and Supplementary Movies 23 ) confirmed that the fences and the hexagonal honeycomb arrays are the side and the top views of the same structure. We propose that when bound to the membrane, the NEC220 oligomerizes into hexagonal honeycomb arrays ( Fig 5d,e , Supplementary Fig. 5c and Supplementary Movie 3 ). UL31/UL31 interactions may contribute to NEC220 coat formation To investigate the ability of the NEC220 to oligomerize, we cross-linked the complex in solution or in the presence of liposomes. In the presence of PC/PS/PA LUVs, the NEC was cross-linked into high-molecular-weight (HMW) oligomers, whereas only individual cross-linked heterodimers were detected in solution ( Fig. 6a ). We saw no cross-linked HMW oligomers in the presence of LUVs suboptimal for binding (PC/cholesterol) ( Fig. 6b ). The stoichiometry of the HMW bands could not be determined, but they contained mostly UL31 and very little UL34 ( Supplementary Fig. 6a,b ), suggesting that the interactions between neighbouring UL31 components may contribute to NEC220 oligomerization ( Fig. 5e ). 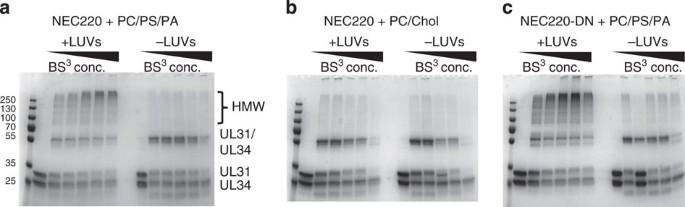Figure 6: NEC220 is cross-linked into high-molecular-weight species in the presence but not absence of acidic LUVs. (a–c) Bis(sulphosuccinimidyl)suberate (BS3) was added at 0, 25, 50, 250, 500, 2500-fold molar excess. Samples were analysed by 12% SDS–PAGE and Coomassie staining. Figure 6: NEC220 is cross-linked into high-molecular-weight species in the presence but not absence of acidic LUVs. ( a – c ) Bis(sulphosuccinimidyl)suberate (BS 3 ) was added at 0, 25, 50, 250, 500, 2500-fold molar excess. Samples were analysed by 12% SDS–PAGE and Coomassie staining. Full size image The non-budding NEC mutant is defective in membrane budding To relate the in vitro observations to the in vivo phenotypes, we tested a NEC mutant known to be deficient in capsid budding. A double point mutation D35A/E37A in UL34 causes a dominant-negative blockage of nuclear egress without affecting formation of the NEC or its localization at the INM [10] . In the presence of this dominant-negative NEC mutant (NEC220-DN), capsids were observed to dock at the INM but the membrane was curved only slightly suggesting a defect in the membrane-deforming activity [10] . Purified NEC220-DN bound membranes in vitro ( Fig. 2a and Supplementary Fig. 2a ) and formed thick clusters on the GUVs but failed to deform GUVs efficiently even after long incubations ( Fig. 3d,g ). In cryoelectron micrographs, the NEC220-DN mutant primarily formed protein spikes on the outer surface of the LUVs ( Fig. 4a,c , and Supplementary Fig. 4c ). Although the outward-facing spikes of the NEC220-DN formed clusters, the typical ‘fence posts’ of the WT NEC220 arranged in the hexagonal arrays were absent, and the clusters were less dense and lacked a regular pattern ( Supplementary Fig. 4c , bottom). In contrast to WT NEC220, protein arrays coating the inner surface of LUVs were rarely observed for mutant NEC220-DN ( Fig 4a,c and Supplementary Fig. 4b,c ). NEC220-DN was cross-linked even more efficiently than the WT NEC220 in the presence of the membrane ( Fig. 6c and Supplementary Fig. 6c,d ), probably because most of NEC220-DN remained primarily on the outside of the LUVs and accessible to the cross-linker ( Fig. 4a,c ). But despite clustering on the membrane surface, the NEC220-DN mutant was clearly deficient in forming the hexagonal arrays. The inability of the NEC220-DN mutant to mediate budding could be due to its inability to oligomerize properly and form the hexagonal arrays, which we think is necessary for membrane deformation. We propose that the non-budding phenotype of the NEC-DN results from a defect in membrane deformation and scission ( Fig. 4d ), linking its in vitro membrane deformation activity with the in vivo budding phenotype. Although the NEC was known to cause vesiculation of the nuclear envelope in transfected cells in the absence of any other viral proteins, it was unclear whether the NEC directly participated in membrane deformation or served to recruit cellular proteins. In this study, we purified recombinant soluble HSV-1 NECs either lacking the TM anchor or containing an anchor mimic and characterized their interactions with model membranes. By reconstituting the budding reaction in vitro entirely from purified NEC and lipids, we establish that the NEC has the intrinsic ability to drive membrane invagination and scission and represents a novel virus-encoded membrane-budding machinery. We found that the soluble NEC220 bound model membranes in the absence of a TM anchor. This binding required a high amount of acidic lipid, at least 40%, and was eliminated in the presence of high salt during co-incubation. This suggested that the recruitment of the soluble NEC220 to membranes required electrostatic interactions. Although in vivo the NEC is anchored to the membrane by means of the TM anchor of UL34, we anticipate that membrane deformation by the NEC may involve substantial contacts between the protein and the membrane beyond mere anchoring. Thus, electrostatic interactions between the NEC and the membrane may yet be important for membrane budding. Electrostatic protein/membrane interactions have been previously observed for other membrane-binding proteins [23] , [24] . Multiple basic residues within residues 186-220 of UL34 may contribute the electrostatic component of membrane binding because the NEC185 binds membranes poorly. Although it is unknown whether residues 186-220 interact with membrane directly, a mutant form of a closely related alphaherpesvirus pseudorabies virus in which UL34 lacks 90 C-terminal residues is nonfunctional despite unimpaired interaction with UL31 (ref. 25 ). The pseudorabies virus NEC containing this truncated UL34 is essentially equivalent to HSV-1 NEC185, and its nonfunctional phenotype could be due to disrupted membrane interactions. After the initial electrostatic attachment, however, the membrane binding of NEC220 is no longer sensitive to salt suggesting that forces other than electrostatic come to dominate binding after attachment. We found that while amino acids 40–50 of UL31 were required for binding to acidic membranes, mutating basic residues within this region did not reduce membrane binding. In the absence of the crystal structure of the NEC, it is unclear whether these residues interact with the membrane directly or influence membrane interaction through an indirect mechanism, for example, by stabilizing other residues in the NEC that directly interact with the membrane. In this latter scenario, single-residue substitutions may not have an effect on the binding ability. More specific explanation of the mutagenesis results awaits the structure of the NEC. The membrane interaction of NEC220 is irreversible suggesting that the initial attachment is followed by oligomerization that results in a tightly bound protein coat that does not dissociate. Using cryo-EM, we observed that incubation of the NEC with LUVs (300–800 nm) leads to the formation of smaller vesicles (100–300 nm) that are coated with the NEC on the inside. Because the NEC is not expected to penetrate the membranes, we infer that the NEC-coated vesicles are the product of completed budding and scission. The individual membrane-bound NEC molecules form spikes that resemble stems topped with spheres ( Fig. 5 ). The spikes form regular hexagonal honeycomb arrays, or coats, that appear as ‘fences’ in side views. The model of the membrane-bound NEC coat is shown in Fig. 5e . In this coat model, UL31 is tentatively assigned to the ‘sphere’ part on the basis of the cross-linking data while UL34 is tentatively assigned to the ‘stem’ part because in full-length NEC, UL34 anchors the complex to the membrane. But, because the precise localization of the two proteins within the membrane-bound NEC spike is unknown, we cannot exclude the possibility that UL31 may also interact with the membrane. Likewise, UL34 may be directly involved in oligomerization: the DN mutations in UL34 appear to interfere with the formation of the hexagonal coat, and residues D35 and E37 of UL34 may be directly involved in the NEC oligomerization. Alternatively, the DN mutations may affect the UL31 oligomerization through an allosteric mechanism. This may explain why in vivo the NEC-DN mutant is deficient in budding despite localizing to the INM. Soluble NEC220 oligomerizes only in the presence of the membrane, suggesting that membrane binding induces a conformational change that exposes the oligomerization surface. The NEC-budding activity in vivo could potentially be controlled through inhibition of oligomerization. The extensive vesiculation of the INM in NEC-transfected cells is not normally observed in infected cells where budding requires the presence of a capsid implying that the intrinsic budding activity of the NEC is suppressed in its absence. In the presence of untagged soluble or membrane-anchored NEC, the budding process occurs very rapidly in vitro . Both soluble and membrane-anchored NECs mediated budding with similar efficiency, ~12–13%. This budding efficiency may appear low compared with the ~70% budding efficiency observed for ESCRT-III using a similar assay [13] ; yet, we do not know what budding efficiency should be expected for NEC under our experimental conditions. Increasing the protein concentration or the incubation time resulted in clusters or aggregates of small vesicles that probably represent budding carried to completion when no ‘mother’ vesicles remain. This observation suggests that the apparent low budding efficiency may be an underestimation, likely because a number of Cascade Blue-containing ILVs are too small to be reliably detected by confocal microscopy. Although we cannot visualize all stages in the NEC-mediated budding process, by analogy with other membrane-budding proteins, we expect that membrane budding by the NEC220 proceeds through a series of steps that begins with membrane binding by the NEC220 and its oligomerization that leads to membrane invagination and is followed by bud formation and, ultimately, scission ( Fig. 4d ). The inward topology of the NEC220-mediated budding and scission observed in vitro resembles capsid budding into the INM during HSV-1 infection and nuclear envelope vesiculation in NEC-transfected cells. While the curvature of the INM is likely neutral or slightly negative, the curvature of the outer surface of the GUVs and especially LUVs is positive. Therefore, when mediating budding of the GUVs or LUVs, the NEC would have to overcome the initial positive curvature, ‘doing extra work’, so to speak, which would not be necessary during budding into the INM. This could explain the flattened surface sometimes generated by the NEC upon binding to GUVs at early time points. To connect further the in vitro observations to the in vivo budding phenotype, we show that a mutant of UL34 that blocks egress in a dominant-negative manner is defective in membrane budding in vitro. This dominant-negative mutant NEC-DN localizes correctly to the INM but is impaired in membrane deformation around the capsid and has a non-budding phenotype [10] . This is consistent with our results showing that the NEC220-DN is impaired in membrane budding in vitro despite being able to interact with LUVs or GUVs. The use of soluble NEC220 and acidic liposomes in reconstitution may appear artificial because in infected and transfected cells, the NEC is membrane-anchored and the INM does not have a high acidic lipid content. Yet, we show that the budding of the acidic GUVs by soluble NEC220 is recapitulated by the budding of the less acidic GUVs by the membrane-anchored NEC220-His, which establishes that our in vitro system adequately models the in vivo budding and can be used as an experimental system for studying the budding mechanism in vitro . Moreover, although the TM of UL34 is essential in vivo , its substitution with the TMs of other nuclear membrane proteins does not affect the function [26] arguing that the primary role of the TM is to anchor the NEC in the INM rather than to participate in membrane budding directly. Based on our results, we propose that the NEC enables budding and scission by a rapid and likely cooperative formation of a coat-like hexagonal array that efficiently scaffolds the membrane from the inside and narrows the neck to the point of scission ( Figs 4d , 5e ). This scission mechanism differs from that of the ESCRT-III proteins, which localize only to the neck but not to the nascent vesicle itself and probably cleave the neck from its exterior end [13] . Energy provided by NEC/membrane and NEC/NEC interactions appears sufficient to drive membrane envelopment. Taken together, our work suggests that the HSV-1 NEC represents the minimal membrane deformation and scission machinery that can function without the need for host factors. Our experiments cannot exclude the possibility that herpesviruses may still recruit cellular factors to regulate nuclear budding in vivo . Recent work has shown that the process of nuclear egress is not unique to herpesviruses and also occurs during the export of large cellular synaptic ribonucleoparticles in Drosophila [27] . Although the cellular protein(s) involved in cellular INM budding have not yet been identified, these may potentially be recruited by herpesviruses. Regardless of which cellular proteins, if any, are necessary for the NEC-mediated nuclear budding, in infected cells nuclear budding is clearly under the control of additional viral proteins. During infection, a virus-encoded protein likely inhibits the budding activity of the NEC until the presence of a capsid relieves this inhibition and allows budding to proceed. The capsid may also specify the size of the budded vesicle; the perinuclear vesicles in NEC-transfected cells, while comparable in size to the perinuclear viral particles in infected cells, are not uniform [11] . This is consistent with our cryo-EM experiments, where the size of the NEC-coated vesicles, which represent the final stage of budding, is not uniform and varies from 100–300 nm. In addition, viral proteins are thought to regulate the deenvelopment step of nuclear egress, which follows budding, whereby the NEC coat has to disassemble to allow the fusion of the primary viral particles with the outer nuclear membrane. Phosphorylation of UL31 by US3 kinase is necessary for the deenvelopment [28] and could, perhaps, enable the disassembly of the NEC coat by weakening the lateral interactions between NEC heterodimers. Interestingly, US3 phosphorylates several residues within the N terminus of UL31 (ref. 28 ) raising the possibility that the phosphorylation status of the N terminus of UL31 may regulate both the budding and the deenvelopment steps of nuclear egress. Many enveloped viruses encode their own membrane deformation proteins—matrix proteins—but most rely on cellular ESCRTs for membrane scission (reviewed in refs 1 , 2 , 3 ). For example, while HIV matrix protein Gag scaffolds the inner surface of the membrane bud, it is insufficient for scission [29] and recruits cellular ESCRT-III proteins, which mediate membrane scission [13] by assembling into a dome-like helical polymer on the inner surface of the neck and constricting it [30] . Nevertheless, several viruses do not require ESCRTs for budding. Budding of influenza virus is ESCRT-independent and is mediated by matrix protein M1, thought to function as a scaffolding protein [31] , and M2, the only known viral scission protein [18] , [31] . Influenza budding is thus accomplished entirely by virus-encoded budding machinery without the need for assistance of host proteins. Budding of flaviviruses [32] and togaviruses [33] is also independent of cellular ESCRT machinery and is thought to be driven entirely by the formation of a virus-encoded outer coat [32] . But the mechanism is topologically opposite to the NEC-budding mechanism because the glycoprotein coat covers the outer surface of the budded virions. Our findings expand the repertoire of ESCRT-independent budding mechanisms. The NEC-budding mechanism is clearly different from those described for other membrane-deforming proteins and may be unique because both bud formation and scission are completed through the formation of an inner scaffold (an inner coat). The idea that membrane deformation and scission by the NEC occurs by a unique mechanism is reinforced by the fact that it is the only currently known viral or cellular protein complex that mediates budding of the nuclear membrane as opposed to cytoplasmic membranes. In biological membranes, lipids are known to segregate into different lipid phases and form microdomains. Differences in lipid composition at the phase boundary can exert the so-called line-tension force capable of driving changes in membrane curvature. Many cellular and viral proteins interact with and manipulate one defined lipid phase, which may cause changes in line tension [31] . For example, protein may induce lipid-phase segregation at the neck of the bud helping create a high-tension lipid environment conducive to membrane scission, a mechanism that has been proposed to play a role in scission mediated by Influenza M2 protein [18] , [31] . Future work will explore lipid requirements of NEC-mediated membrane budding and the possibility that NEC-mediated changes in line tension may provide the driving force for alterations in membrane curvature. The essential function in the viral infectious cycle provided by the NEC provides new targets for the development of antiviral therapeutics. In particular, strategies to block the NEC coat assembly may lead to successful therapeutic interventions based on blocking the capsid egress from the nucleus. Plasmid cloning Plasmids encoding HSV-1 strain F UL31 (GenBank accession number ADD60001.1 ) with domain boundaries 1-306 (full-length UL31, pKH90), 51-306 (UL31Δ50, pKH86) or 41-306 (UL31Δ40, pJB41) were generated by PCR with primers (full-length forward 5′-AGCA GGATCC TATGACACCGACCCCCAT-3′; Δ50 forward 5′-AGCA GGATCC CAGGAGCTGTGTTTACAC-3′; Δ40 forward 5′-AAAAAA GGATCC CGGAAGAGCCTGCCG-3′; reverse 5′-AAATG CGGCCGC TTACGGCGGAGGAAACTC-3′) containing BamHI and NotI restriction sites (underlined). Fragments were cloned into the prokaryotic expression vector pET24b (Invitrogen) modified to include a sequence encoding a His6-SUMO tag followed by a PreScission cleavage site. Plasmids encoding HSV-1 strain F UL34 (GenBank accession number ADD60035.1 ) with domain boundaries 1-220 (UL34(1-220), pJB02) and 1-185 (UL34(1-185), pJB03) were generated by PCR with primers (forward 5′-AAAAAA GTCGAC CTATGGCGGGACTGGGCAAG-3′; reverse 220 5′-AAAAAA GCGGCCGC CTTCAGTCCCCCCTGGCCC-3′; reverse 185 5′- AAAAAA GCGGCCGC CTTCAGGCGGCGCGGCACA-3′) containing Sal I and Not I restriction sites (underlined). Fragments were cloned into pGEX-6P1 (GE Healthcare) that encodes an N-terminal GST-tag followed by a PreScission cleavage site. Site-directed mutagenesis of the double, triple or quadruple mutations in UL31 (R49A/K50 (pJB27), R41S/K42S (pJB48), R49S/K50S (pJB51), L44S/P45T/P46T (pJB50), L44S/A48S (pJB47), and R41S/K42S/R49S/K50S (pJB54)) and UL34 (D35A/E37A (pJB21)) was performed using the splicing-by-overlap-extension PCR [34] using primers (R49A/K50 forward 5′-GAGCCTGCCGCCTCACGCCGCCGCACAGGAGCTGTGTTTACACGAG-3′; R49A/K50A reverse 5′-CTCGTGTAAACACAGCTCCTGTGCGGCGGCGTGAGGCGGCAGGCTC-3′; R41S/K42S forward 5′-GGTGCGTCGGGCCTCCAGCAGCAGCCTGCCGCCTCACG-3′; R41S/K42S reverse 5′-CGTGAGGCGGCAGGCTGCTGCTGGAGGCCCGACGCACC-3′; R49S/K50S forward 5′-GAGCCTGCCGCCTCACGCCAGCAGCCAGGAGCTGTGTTTACACGAG-3′; R49S/K50S reverse 5′-CTCGTGTAAACACAGCTCCTGGCTGCTGGCGTGAGGCGGCAGGCTC-3′; L44S/P45T/P46T forward 5′-GGCCTCCCGGAAGAGCAGCACGACTCACGCCCGCAAACAGG; L44S/P45T/P46T reverse 5′-CCTGTTTGCGGGCGTGAGTCGTGCTGCTCTTCCGGGAGGCC-3′; L44S/A48S forward 5′-GGCCTCCCGGAAGAGCAGCCCGCCTCACAGCCGCAAACAGG-3′; L44S/A48S reverse 5′-CCTGTTTGCGGCTGTGAGGCGGGCTGCTCTTCCGGGAGGCC; R41S/K42S/R49S/K50S forward and reverse primers for R49S/K50S on R41S/K42S template; D35A/E37A forward 5′-GGGCGGGGCCGGGGCGGCGGGCCCC-3′; D35A/E37A reverse 5′-GGGGCCCGCCGCCCCGGCCCCGCCC-3′). Protein purification Plasmids encoding UL31 or UL34 were co-transformed into E . coli BL21(DE3) Rosetta cells (Novagen) and expressed at 18 °C for 16 h after induction with 0.3 mM IPTG. All purification steps were performed at 4 °C. All complexes were purified in lysis buffer (50 mM HEPES pH 7.0, 500 mM NaCl, 10% glycerol and 1 mM TCEP) unless noted otherwise. Cells were resuspended in lysis buffer in the presence of complete protease inhibitor (Roche) and lysed using French Press. The cleared cell lysate was first passed over a Ni-NTA sepharose (GE Healthcare); the column was washed with lysis buffer containing 20–40 mM imidazole, and bound proteins were eluted with lysis buffer containing 250 mM imidazole and loaded onto a glutathione sepharose to obtain the NEC free from excess His6-SUMO-UL31. After washing with lysis buffer, His6-SUMO and GST tags were cleaved on the glutathione sepharose column for 16 h using PreScission protease produced in house using a GST-PreScission fusion protein expression plasmid. Cleaved proteins were eluted from the GSH column with lysis buffer. Protein-containing fractions were diluted to obtain 50 mM NaCl and applied onto a cation exchange column (HiTrap SP XL, GE Healthcare). The NEC was eluted using a NaCl gradient. As the final purification step, proteins were purified by size-exclusion chromatography using a Superdex 75 column (GE Healthcare) equilibrated with 20 mM HEPES, pH 7.0, 100 mM NaCl, 1 mM TCEP. The column was calibrated using blue dextran (~2,000 kDa), conalbumin (75 kDa), carbonic anhydrase (29 kDa), ribonuclease A (13.7 kDa) and aprotinin (6.5 kDa). The NEC complexes were purified to homogeneity as assessed by 12% SDS–PAGE and Coomassie staining. Fractions containing the NEC were concentrated up to 80 μM (~5 mg ml −1 ) and stored at −80 °C to avoid aggregation and degradation at 4 °C. Protein concentration was determined by absorbance measurements at 280 nm. The typical yield was 1.5 mg l −1 LB culture. SNAP-tagged full-length UL31 was expressed using pET28a vector that was modified to contain a SNAP-tag (New England Biolabs) at the C-terminal end of the UL31 insert (gift from A. Rodal, Brandeis University). Expression and purification were performed as for the NEC220 in the same buffers until the gel filtration step. Before applying the complex onto the S75 column, it was incubated with SNAP surface 488 dye (New England Biolabs) at a 1:2 molar ratio in the presence of 1 mM DTT for 16 h at 4 °C. Protein complexes containing an additional C-terminal His-tag on UL34, to mimic the transmembrane region, were purified as above. Multi-angle light scattering For SEC-coupled multi-angle light scattering, 200 μg of the NEC at 1 mg ml −1 were injected onto a Superdex S75 column (GE Healthcare), equilibrated in 20 mM HEPES pH 7.0, 100 mM NaCl, 1 mM TCEP overnight at 4 °C. The chromatography system was connected in line to a DAWN Heleos II light-scattering instrument equipped with a 658-nm laser and Optilab T-rEX interferometric refractometer (Wyatt Technology). Data were analysed with ASTRA 6 software (Wyatt Technology), yielding the molar mass and mass distribution (polydispersity) of the sample. Monomeric and dimeric BSA was used for normalization of the light-scattering detectors and data quality control. CD spectroscopy The NEC220 (5 μM) was exchanged into CD buffer (20 mM sodium phosphate buffer pH 8.0, 100 mM NaF). The far-ultraviolet CD spectrum of the protein was then measured at 20 °C on a JASCO-810 spectropolarimetre equipped with Peltier cell (Elfin model ELDC5D4) and a 1 cm quartz cuvette using 50 nm sec −1 scan speed, 1-nm band pass and 1-s response time. For each sample, three scans were collected and averaged, a buffer blank spectrum was subtracted and the sample was processed for noise elimination. Measurements are presented in units of mean residual ellipticity (θ). The secondary structure content was calculated from the CD spectra using CDSSTR and reference set 7 on the Dichroweb server. Thermal denaturation was monitored at 222 nm (θ 222 ) with simultaneous monitoring of the temperature at a heating and cooling rate of 2.0 °C min −1 . The temperature reading was taken at the heating/cooling disk that holds the measurement cuvette. Denaturation and renaturation spectra were averaged from two independent measurements. The first derivatives of the denaturation curves were calculated using ORIGIN version 7.0 and fitted to a single Lorentzian line. The melting temperature T m was determined from the maximum point of the first derivative. Measurements were taken every 2 °C with a 1-s response time. Liposome preparation POPC, POPS or POPA were dissolved in chloroform at 10 mg ml −1 final concentration, mixed in various ratios and dried into a layered film in a glass vial under vacuum or argon. The lipid films were further dried in a vacuum oven for 30 min and then hydrated in 20 mM Na-HEPES, pH 7.0, 250 mM NaCl, 1 mM TCEP at 20 °C for 4–16 h. Hydrated lipids were extruded through a 800, 400 and/or 100-nm filter using the Avanti Polar Mini-Extruder, per the manufacturer’s protocol. LUVs were separated from debris in a tabletop centrifuge at 18,000 g for 10 min at room temperature. LUVs were stored at 4 °C and used within 1 week. For use in the co-sedimentation assay, lipids were dried as above and hydrated for 2 h at 37 °C to yield MLVs. Hydrated lipids were vortexed, stored at 4 °C for 16 h and used immediately. GUVs were prepared as described previously [17] . Briefly, lipids were mixed in a molar ratio of 58% POPC/19.5% POPS/19.5%POPA/3% POPE-Atto594 or 58% POPC/11% POPE/9% POPA/9% POPS/5% cholesterol/5% DGS-NTA/3% POPE-Atto594 of a vacuum-dried lipid mixture, dissolved in dichloromethane:methanol (8:2, v/v, final total lipid concentration 10 mg ml −1 ), were spread on the surface of an ITO-covered slide and dried in a vacuum oven for 30 min. A vacuum-greased O-ring was placed around the lipid mixture. An AC field (sinusoidal wave function with a frequency of 8 Hz and amplitude of 2 V) was applied using the Vesicle Prep Pro (Nanion Technologies) before adding 280 μl of 300 mM sucrose dissolved in 5 mM Na-HEPES, pH 7.5. After a 3-minute rise step, a second ITO-covered slide was used to cover the lipid mixture, and a 2-h swell and a 5-minute fall step completed the protocol. The GUVs were stored at 4 °C and used within 1 day. GUVs were diluted with 20 mM Na-HEPES, pH 7.0, 20 mM NaCl in a 1:10 ratio before imaging. GUVs prepared using this method typically had a diameter of 3–10 μm. Coflotation assay The NEC-membrane interaction was tested using coflotation as described previously [35] . Briefly, the NEC (3 μg) was incubated with or without LUVs (100 nm) at 37 °C for 1 h in 50 μl PBS. NaCl was added to 1 M concentration to reduce nonspecific protein–membrane interactions, and samples were incubated for 15 min at 37 °C. Sucrose was added to a final concentration of 40% in a 500 μl volume. Samples were placed at the bottom of a 5-ml centrifugation tube (Beckmann) and overlaid with 4 ml 25% sucrose and 500 μl 5% sucrose in PBS. The samples were next centrifuged in a Beckman SW-55 Ti rotor at 246,000 g for 3 h at 4 °C, and 1 ml fractions were collected beginning at the top. The fractions analysed by 12% SDS–PAGE and Western Blot using polyclonal anti-UL31 or anti-UL34 antibodies. Co-sedimentation assay A quantity of 3 μg of protein was centrifuged at 16,000 g for 20 min at 4 °C to get rid of nonspecific aggregates and debris. The supernatant was incubated with or without 15 μg of freshly prepared MLVs at 20 °C for 30 min. The samples were centrifuged again at 16,000 g for 20 min at 4 °C. Aliquots of input fractions, protein/MLV pellet, and protein supernatant were analysed by 12% SDS–PAGE and Coomassie staining. The amount of protein that pelleted with MLVs was determined by densitometry analysis of gels imaged using GBox (Syngene) and quantified using manufacturer’s software GeneTools. For each protein, band intensities of the pelleted protein were integrated and expressed as a percentage of the total integrated intensity of all bands, that is, protein pelleted with MLVs plus un-pelleted protein. Each experiment was done in triplicate, and the average value and the standard error of measurement is reported. GUV deformation assay A volume of 10 μl of GUVs containing POPE-Atto594 at a concentration of 0.2 μg μl −1 were mixed with a final concentration of 0.8 μM NEC200-SNAP488 and incubated for 5 min at 20 °C or 30 min on ice, respectively. The total volume of the samples during imaging was 100 μl and imaging was performed in an 8-well (or 96-well) chambered coverglass. Images were acquired using a Spinning Disk Confocal Microscope at the Brandeis University CLEM facility (Zeiss AxioObserver) or at the Department of Pathology at Tufts University School of Medicine (Zeiss Axiovert 200). Additional images were acquired using a Nikon A1R Confocal microscope at the Tufts Imaging facility of the Center for Neuroscience Research at Tufts University School of Medicine and at the Confocal and Light Microscopy Core Facility at Dana Farber Cancer Institute. In all cases, a × 100 oil immersion lens was used. Image analysis was performed using ImageJ [36] . Where applicable, 0.2 mg ml −1 Cascade Blue Hydrazide (Life Technologies) was added to diluted GUVs. Quantification was performed by counting all vesicles in 17 random frames of each sample. The experiments were repeated twice independently. The number of vesicles counted in total are as follows: no protein (104, 111), NEC220 (83, 75, 119), NEC220-DN (77, 136), NEC220-His (67, 86, 109). Cryoelectron microscopy Holey carbon Quantifoil copper grids (R2/2, 200 mesh, Quantifoil Micro Tools) were glow discharged for 45 s at −20 mA, mounted on a forceps and loaded into a Gatan CP3 plunger (Gatan). A volume of 10 μl of a 1:1 mixture of 400-nm and 800-nm LUVs were mixed with 30 μl buffer or protein (NEC220 or NEC220-DN mutant) and incubated on ice. After 30 min, 3 μl of sample were pipetted onto the grid, mixed with 1 μl of fivefold concentrated 10 nm colloidal gold (Sigma-Aldrich) that was coated with BSA [37] , blotted for 4 s from both sides and vitrified by rapidly freezing in liquid ethane at −180 °C. Cryo samples were stored in liquid nitrogen until transferred to a Tecnai F20 transmission electron microscope (FEI) via a cryo holder (Gatan). The microscope was operated in low dose mode at 200 keV using SerialEM [38] and images were recorded with a 4k × 4k charge coupled device camera (Ultrascan, Gatan) at 19,000 (pixel size: 0.946 nm) or 29,000-fold magnification (pixel size: 0.632 nm). 2D cryo-EM images were recorded at defocus values of −4 to −8 μm and an electron dose of 15 e/Å 2 . For 2D averaging, 262 NEC220 hexamers were selected from a micrograph showing a ring-like array of NEC220 ( Fig. 4b ) and averaged with or without imposing sixfold symmetry with the software PEET (particle estimation for electron tomography [39] ). Single axis cryo-ET was used to generate 3D EM data: tilt series were acquired by stepwise tilting the sample from −60 to +60° in 1.5–2.5° increments and recording 60–100 images. Electron micrographs were recorded at 19,000-fold magnification with −6 to −8 μm defocus. The accumulative electron dose was restricted to ~100 e/Å 2 to minimize radiation damage. The IMOD software package [40] was used for tomogram reconstruction from the recorded tilt series. For 3D (subtomogram) averaging, 240 NEC220 hexamers (identified as circles in top views) were selected from a tomogram of LUVs with NEC220 ( Supplementary Movie 1 ) and averaged with and without imposing sixfold symmetry in 3D with the software PEET [39] . Using the 0.5 correlation score criterion of the Fourier Shell Correlation [41] the resolution of the sixfold symmetric average was estimated to be 3.5 nm. Protein cross-linking and western blots A volume of 6 μg protein was incubated with or without 50 μg of LUVs (100–800 nm) for 1 h at 37 °C. BS 3 cross-linker (Thermo Scientific) was added at 0, 25, 50, 250, 500 and 2500-fold molar excess and the samples were incubated for 30 min at room temperature. The reaction was stopped by adding Tris–HCl, pH 8.0 to a final concentration of 50 mM, followed by incubation at room temperature for 15 min. The samples were analysed by 12% SDS–PAGE and either Coomassie staining or western blots. For western blots, the nitrocellulose membranes were incubated with either the polyclonal anti-UL31 rabbit antibody at a 1:10,000 dilution or a polyclonal anti-UL34 chicken antibody at a 1:1,000 dilution (see antibody details below). Following incubation in the primary antibodies for 1 h at room temperature, the blots were incubated in goat anti-rabbit or anti-chicken IgG horseradish peroxidase conjugated secondary pAb (1:8,000 dilution) for 1 h and developed using the Pierce Western Pico chemiluminescence kit. Antibodies Polyclonal rabbit antibody against HSV-1 UL31 was generated by Cocalico Biologicals using purified full-length UL31 as the immunogen. UL31 precipitated over the course of purification but could be used for antibody production. Polyclonal chicken antibody against HSV-1 UL34 was a gift from R. Roller (University of Iowa). How to cite this article: Bigalke, J. M. et al. Membrane deformation and scission by the HSV-1 nuclear egress complex. Nat. Commun. 5:4131 doi: 10.1038/ncomms5131 (2014).